Antigen capture and archiving by lymphatic endothelial cells following vaccination or viral infection Antigen derived from viral infections with influenza and vesicular stomatitis virus can persist after resolution of infection. Here we show that antigen can similarly persist for weeks following viral challenge and vaccination. Antigen is captured by lymphatic endothelial cells (LECs) under conditions that induce LEC proliferation. Consistent with published data showing that viral antigen persistence impacts the function of circulating memory T cells, we find that vaccine-elicited antigen persistence, found on LECs, positively influences the degree of protective immunity provided by circulating memory CD8 + T cells. The coupling of LEC proliferation and antigen capture identifies a mechanism by which the LECs store, or ‘archive’, antigens for extended periods of time after antigen challenge, thereby increasing IFNγ/IL-2 production and enhancing protection against infection. These findings therefore have the potential to have an impact on future vaccination strategies and our understanding of the role for persisting antigen in both vaccine and infectious settings. In conjunction with generating robust, enduring cellular immunity, antigen derived from infectious agents often persists for an extended period of time after the infection is cleared from the host [1] , [2] , [3] , [4] , [5] . Flu antigens persist in the lung-draining lymph nodes (LNs) [5] , [6] , [7] and within the respiratory tract [1] , [3] well after the clearance of the primary infection. Although it is clear that the maintenance of CD8 + T-cell memory does not require the presence of antigen over time [8] , [9] , it is also clear that antigen persistence after viral infections can have an overall positive influence on the maintenance of protective T-cell immunity. Flu-related antigens within the lung-draining nodes or inducible bronchus associated lymphoid tissue periodically stimulate circulating memory cells to proliferate and differentiate into more effector-like cells [2] , [3] , [5] , [10] . The proliferation that accompanies this process serves to increase the concentration of viral-specific effector T cells within the local tissue, enhancing protective immunity by initiating a rapid response in situ to rechallenge [1] , [5] . This type of antigen persistence is in sharp contrast to the high antigen loads resulting from chronic viral infections, which typically produce a hypo-responsive memory T-cell pool [11] . Thus, the functional significance of both persisting and chronic viral antigen are well established. Considerably less clear are the precise cellular locations of persisting antigen that can stimulate antigen-specific CD8 + T cells. Follicular dendritic cells (FDCs) are a non-haematopoietic cell (CD45 − ) characterized by gp38 and CD21/35 expression, the latter (complement receptors 1 and 2) being important for the function of FDCs in holding antigen/antibody complexes for extended periods of time [12] . Historically, FDCs have been documented as a source of persisting antigen [13] associated with antigen presentation to B cells and helper T cells. Specifically, persisting antigen was thought to be part of the process of follicle maturation and B-cell memory formation where antigen is hidden within the tendrils of the FDC for later presentation to memory B cells [14] . More recently, an elegant imaging study showed the mechanism by which antigen/antibody complexes are maintained for long periods of time, being continually internalized and resurfaced on the FDC [12] . Although FDCs have been long thought to be the CD45 − cell associated with all reservoirs of persisting antigen, there are other CD45 − stromal subsets that line the subcasular sinus (lymphatic endothelial cells (LECs)), blood vessels (blood endothelial cells), or act as conduits for the migration and trafficking of T cells and dendritic cell (DCs) (fibroblastic reticular cells) within the LN or white pulp. Besides lining the lymph vessels, LECs project into the interfollicular ridges and T-cell zones, and are important for LN structure as well as some antigen presentation and DC cell trafficking [15] , [16] , [17] , [18] , [19] . Most stromal cells express Toll-like receptors (TLRs) and may play a role during inflammatory responses as well [17] . Although unique mechanisms behind how FDCs hold onto whole antigen and cooperate with B cells were recently identified [12] , no reports to date have established whether stromal cell types other than FDCs can facilitate antigen persistence following infection or vaccination. Here we demonstrate that both viral challenge and subunit vaccination induce antigen to persist in the host for times extending well beyond the peak of the T-cell response to the immunologic challenge. Surprisingly, we found that the persisting antigen resides on LECs, a stromal cell subset not previously characterized for antigen capture and persistence. Perhaps most significant is our observation that antigen persistence is dependent not specifically on T or B cells, but instead on LEC proliferation in the context of a productive immune response. The coupling of LEC proliferation and antigen capture identifies a previously unappreciated mechanism by which the stroma in secondary lymphoid tissue maintains antigens against which a robust response has been initiated, in effect ‘archiving’ these antigens for periods of time lasting well after the peak of the normal immune response. Consequently, the presence of archived antigen on LECs results in a memory CD8 T-cell pool with increased effector function and protective capacity. Thus, given the functional consequences of antigen persistence on T cells after viral infection [1] , [2] , [3] , [4] , [5] and vaccination, as we show here, these results are significant as the first report to identify LEC involvement in this process. Antigen persists following viral infection Previous studies have shown that viral antigens can be detected in mice well after the peak of the CD8 T-cell response and clearance of the infection. We obtained similar results using Vaccinia virus (VV) as a model viral challenge. Persistence of viral antigen was observed by using the transfer of carboxyfluorescein succimidyl ester (CFSE) labelled transgenic T cells (OT1 transgenic cells, specific for the SIINFEKL peptide derived from ovalbumin) at various time points after infectious challenge with an ovalbumin-expressing strain of VV (VV-ova). The proliferation of the transferred cells, as gauged by the loss of CFSE fluorescence, was used as a functional readout for the presence or absence of persisting antigen. Compared with infection with an ovalbumin-expressing strain of Listeria monocytogenes (LM, LM-ova), which resulted only in a brief period of antigen persistence [20] , VV infection resulted in antigen persistence ( Fig. 1 ) long after (>30 days) the endogenous T-cell response had peaked and declined to <1% of the total CD8 + T cells. This time frame of VV antigen persistence is similar to that observed for flu antigens [1] , [3] , [5] . We conclude from these data that virus-associated antigen persists for periods of time well after clearance of infection, and the magnitude of antigen persistence is sufficient to result in substantial proliferation of naive antigen-specific CD8 + T cells in the host. 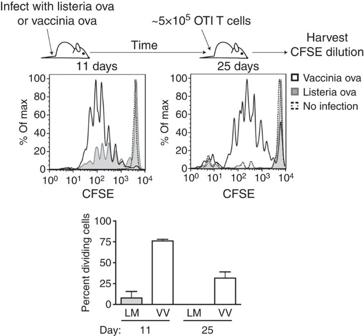Figure 1: Antigen persists following infection with VV. Mice were challenged with either VV-ova or LM-ova. CFSE-labelled, congenically different (CD45.1+) OT1 T cells were transferred on day 8 or day 22 after challenge. Three days post T-cell transfer, mice were killed and single-cell suspensions were generated from each spleen. Cells were positively gated for CD8 and CD45.1, and T-cell proliferation was assessed by CFSE dilution by flow cytometery. The per cent of OT1 cells that are dividing was calculated as described in the Methods. Data are representative of two experiments with at least three mice per group with similar results. Error bars represent the s.e.m. Figure 1: Antigen persists following infection with VV. Mice were challenged with either VV-ova or LM-ova. CFSE-labelled, congenically different (CD45.1 + ) OT1 T cells were transferred on day 8 or day 22 after challenge. Three days post T-cell transfer, mice were killed and single-cell suspensions were generated from each spleen. Cells were positively gated for CD8 and CD45.1, and T-cell proliferation was assessed by CFSE dilution by flow cytometery. The per cent of OT1 cells that are dividing was calculated as described in the Methods. Data are representative of two experiments with at least three mice per group with similar results. Error bars represent the s.e.m. Full size image Antigen persists following subunit vaccination To date, all model systems in which antigen persistence has been described use a viral challenge. However, vaccinia stimulates many different inflammatory pathways and expresses many different antigens. To simplify, we used one antigen and one TLR agonist along with a DC activator, anti-CD40, to be able to understand the mechanism by which antigen persists. We [21] , [22] , [23] , [24] , [25] , [26] , [27] , [28] and others [29] , [30] have published extensively on this TLR/αCD40 vaccination method. The reasoning behind examining antigen persistence to this particular vaccine was twofold. First, its capacity to elicit protective cellular immunity and its underpinning molecular mechanisms, are well established [21] , [22] , [23] , [24] , [25] , [26] , [27] , [28] . Second, the magnitude of the T-cell response (CD4 and CD8) following combined TLR/CD40 vaccination is comparable to that observed following model infections such as vaccinia (10–25% of the total T-cell population end up as antigen-specific CD4 or CD8 T cells [21] , [22] , [23] , [24] , [25] , [26] , [27] , [28] , [29] , [30] , [31] ). Mice were immunized with ovalbumin in the context of combined αCD40/polyI:C and at indicated time points after immunization, OT1 T cells were transferred and their proliferation was assessed as an indicator of antigen persistence. As with viral challenge, antigen was not cleared rapidly post immunization, but instead was retained in the LN for at least 3–4 weeks ( Fig. 2a ). Antigen persistence was not specific to ovalbumin because a similar amount of T-cell proliferation was observed after immunization with HSV glycoprotein B (HSVgB) and transfer of T cells from the gBT-1 T-cell receptor (TCR) transgenic (specific for the SSIEFARL epitope from HSVgB) ( Fig. 2b ). Persistence was also not specific to the use of a particular TLR agonist or the use of anti-CD40 in the adjuvant as it was observed following TLR1/2 agonist (Pam3CSK4)/anti-CD40 ( Fig. 2c ) or TLR7 agonist–antigen conjugate (3M019) [32] , [33] vaccination ( Fig. 2d ). Thus, similar to viral challenge, immunization with a spectrum of vaccine adjuvants and antigens results in antigen persistence within the secondary lymphoid tissue. 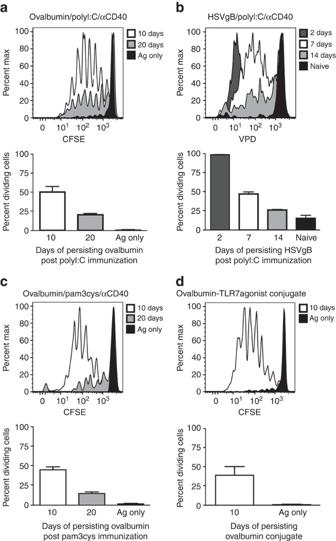Figure 2: Antigen persists following subunit vaccination. (a) Mice were immunized with 100 μg of ovalbumin+50 μg of polyI:C+50 μg of αCD40 or with ovalbumin antigen alone (Ag only). Ten or 20 days post immunization, CFSE-labelled, congenically labelled OT1 T cells were transferred into immunized mice and their division in the spleen assessed 3 days later as inFig. 1. (b) Similar toa, except using 50 μg of whole HSVgB protein as the antigen and VPD-labelled HSVgB-specific TCR transgenic, gBT, as the transferred T cells. (c) Similar toa, except using 25 μg pam3CSK4 as the adjuvant. (d) Mice were immunized subcutaneously with 50 μg of a TLR7 agonist conjugated to ovalbumin. Antigen persistence was measured by proliferation of transferred OT1 cells in the draining LN as ina. The average per cent of dividing cells and s.e.m. of all mice in each group, calculated as described in the Methods, are shown for each plot. Data are representative of two experiments with at least three mice per group with similar results. Error bars represent the s.e.m. Figure 2: Antigen persists following subunit vaccination. ( a ) Mice were immunized with 100 μg of ovalbumin+50 μg of polyI:C+50 μg of αCD40 or with ovalbumin antigen alone (Ag only). Ten or 20 days post immunization, CFSE-labelled, congenically labelled OT1 T cells were transferred into immunized mice and their division in the spleen assessed 3 days later as in Fig. 1 . ( b ) Similar to a , except using 50 μg of whole HSVgB protein as the antigen and VPD-labelled HSVgB-specific TCR transgenic, gBT, as the transferred T cells. ( c ) Similar to a , except using 25 μg pam3CSK4 as the adjuvant. ( d ) Mice were immunized subcutaneously with 50 μg of a TLR7 agonist conjugated to ovalbumin. Antigen persistence was measured by proliferation of transferred OT1 cells in the draining LN as in a . The average per cent of dividing cells and s.e.m. of all mice in each group, calculated as described in the Methods, are shown for each plot. Data are representative of two experiments with at least three mice per group with similar results. Error bars represent the s.e.m. Full size image Persistence influenced by antigen dose and inflammatory stimuli With this reductionist model in hand, we next examined what aspects of the combined adjuvant were required to result in persistence of the antigen past the peak of the endogenous T-cell response. Consistent with the results from the TLR7 conjugate vaccine, we observed that antigen persistence was independent of the anti-CD40 stimulation but dependent on the pro-inflammatory (TLR agonist) portion of the vaccine adjuvant ( Fig. 3a ). This was also true of agonists for TLR2 ( Supplementary Fig. 1 ). In addition, antigen dose correlated with the length of time the antigen persists ( Fig. 3b ), and surprisingly small amounts of polyI:C (0.5 μg) ( Fig. 3c ) were sufficient to induce persistence of minimal amounts of antigen (10 μg). PolyI:C is also an agonist for Mda5 [34] , [35] and induces T-cell responses independent of TLR3. This suggests that inducing antigen persistence may be more broadly applied to innate receptors in general and is not unique to the TLRs. 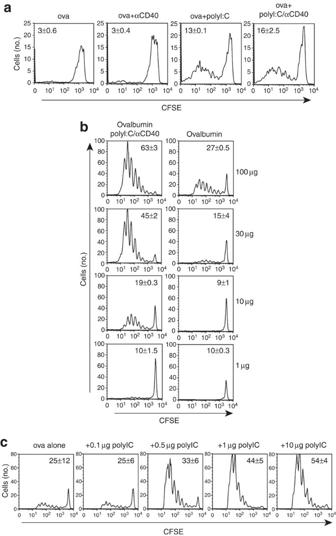Figure 3: Antigen persistence is dependent on innate receptor stimulation and is influenced by antigen dose. (a) Mice were immunized intraperitoneally with 10 μg of ovalbumin in conjunction with either anti-CD40, polyI:C, or both. Six days post immunization, OT1 T cells were CFSE labelled, transferred and their division was assessed 3 days later as inFig. 2a. (b) Mice were immunized with the indicated amount of ovalbumin alone or with 50 μg of polyI:C and 50 μg of anti-CD40. OT1 division was visualized as ina. (c) Mice were immunized with 10 μg of ovalbumin and the indicated amount of polyI:C and OT1 division was assessed as ina. Data are representative of two experiments with at least three mice per group with similar results. Figure 3: Antigen persistence is dependent on innate receptor stimulation and is influenced by antigen dose. ( a ) Mice were immunized intraperitoneally with 10 μg of ovalbumin in conjunction with either anti-CD40, polyI:C, or both. Six days post immunization, OT1 T cells were CFSE labelled, transferred and their division was assessed 3 days later as in Fig. 2a . ( b ) Mice were immunized with the indicated amount of ovalbumin alone or with 50 μg of polyI:C and 50 μg of anti-CD40. OT1 division was visualized as in a . ( c ) Mice were immunized with 10 μg of ovalbumin and the indicated amount of polyI:C and OT1 division was assessed as in a . Data are representative of two experiments with at least three mice per group with similar results. Full size image Antigen persists independent of FDCs or B cells, or CD4 help FDCs are a radio-resistant stromal cell subset that can capture and harbour antigen over extended periods of time [1] , [12] , [13] , [14] , [36] . The mechanism by which FDCs hold antigen is largely through antigen/antibody complexes and their interaction with CR2 (CD21) [12] , [37] , [38] , [39] , [40] . As such, we expected that if antigen persistence following viral infection or combined TLR/CD40 vaccination was dependent on this mechanism, then antigen persistence would be compromised in a CR2-deficient host. However, antigen persistence was largely intact in a CR2-deficient mouse following vaccination ( Fig. 4a ). Furthermore, in hosts with either limited (hen egg lysozyme-specific B-cell receptor transgenic, MD4) or absent (μMT) B-cell repertoires we found no defect in the ability to retain antigen ( Fig. 4b,c ). As FDCs are absent from B-cell-deficient mice [41] , [42] and complement receptors are necessary for FDC antigen capture [12] , [37] , [38] , [39] , [40] , this further diminishes a potential role for FDCs in antigen persistence. Using a mouse deficient for major histocompatibility complex (MHC) class II, we also confirmed that CD4 T-cell help was dispensable for antigen persistence ( Fig. 4d ). Collectively, these data are consistent with the conclusion that antigen persistence can occur independent of CD4 + T cells, B cells, FDCs, antibody production or antigen–antibody complexes. 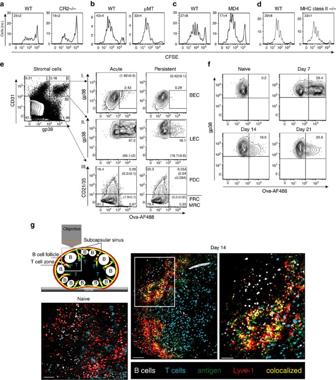Figure 4: LECs capture persisting antigen. (a) Experiments performed as inFig. 2a, where Cr2−/−mice, (b) μMT mice, (c) MD4 mice, or (d) MHC class II−/−mice were assessed for their ability to retain antigen. The average per cent dividing cells and s.e.m. of all mice in each group were calculated as described in the Methods. (e) Mice were injected subcutaneously with 20 μg of ovalbumin conjugated to Alexa Fluor 488, 2 μg polyI:C and 2 μg anti-CD40. Post immunization, mice were killed and draining LNs harvested and prepared, and stained as described in the Methods. Cells shown are CD45−. Arrows indicate which numbered quadrant in the left-most dot plot is being analysed in the same numbered column of plots on the right to visualize fluorescent antigen on (I) Fibroblastic reticular cells (FRC), FDC, or marginal reticular cells (MRC); (II) LECs; or (III). Blood Endothelial Cells (BECs) 1 day (acute) or 6 days (persistent) post immunization. Experiments inewere repeated (10+ times) with at least three mice per group with similar results. Numbers not in parentheses show the per cent of cells with the region in that plot. Numbers in parentheses show the average per cent and s.e.m. of the per cent of cells within the region calculated from all mice in each group. (f) Mice were immunized with 10 μg of fluorescently labelled ovalbumin, 2 μg of polyI:C and 2 μg of αCD40 subcutaneously as ineand draining LN removed, prepared and stained as inaon days 7, 14 or 21 post immunization. (g) Mice were injected in the footpad with fluorescent antigen as inf. Thirteen days later, T cells and B cells labelled with VPD or CMTMR, respectively, were transferred i.v. into immunized mice and anti-Lyve-1 antibody (Alexa Fluor 647) was injected in the footpad. Twelve to 18 h after transfer, mice were killed and popliteal LNs were imaged by multi-photon microscopy as described in Methods. Scale bar, 70 μm in naive, 100 μm in Day 14 and 50 μm in the Day 14 zoomed in box. Imaging experiments ingwere repeated twice with similar results. Figure 4: LECs capture persisting antigen. ( a ) Experiments performed as in Fig. 2a , where Cr2 −/− mice, ( b ) μMT mice, ( c ) MD4 mice, or ( d ) MHC class II −/− mice were assessed for their ability to retain antigen. The average per cent dividing cells and s.e.m. of all mice in each group were calculated as described in the Methods. ( e ) Mice were injected subcutaneously with 20 μg of ovalbumin conjugated to Alexa Fluor 488, 2 μg polyI:C and 2 μg anti-CD40. Post immunization, mice were killed and draining LNs harvested and prepared, and stained as described in the Methods. Cells shown are CD45 − . Arrows indicate which numbered quadrant in the left-most dot plot is being analysed in the same numbered column of plots on the right to visualize fluorescent antigen on (I) Fibroblastic reticular cells (FRC), FDC, or marginal reticular cells (MRC); (II) LECs; or (III). Blood Endothelial Cells (BECs) 1 day (acute) or 6 days (persistent) post immunization. Experiments in e were repeated (10+ times) with at least three mice per group with similar results. Numbers not in parentheses show the per cent of cells with the region in that plot. Numbers in parentheses show the average per cent and s.e.m. of the per cent of cells within the region calculated from all mice in each group. ( f ) Mice were immunized with 10 μg of fluorescently labelled ovalbumin, 2 μg of polyI:C and 2 μg of αCD40 subcutaneously as in e and draining LN removed, prepared and stained as in a on days 7, 14 or 21 post immunization. ( g ) Mice were injected in the footpad with fluorescent antigen as in f . Thirteen days later, T cells and B cells labelled with VPD or CMTMR, respectively, were transferred i.v. into immunized mice and anti-Lyve-1 antibody (Alexa Fluor 647) was injected in the footpad. Twelve to 18 h after transfer, mice were killed and popliteal LNs were imaged by multi-photon microscopy as described in Methods. Scale bar, 70 μm in naive, 100 μm in Day 14 and 50 μm in the Day 14 zoomed in box. Imaging experiments in g were repeated twice with similar results. Full size image Antigen persists on LECs An important role for radio-resistant cells in holding antigen following viral infection was shown in a previous study [1] , although the precise radio-resistant stromal cell subset was never specifically identified. Using established markers ( Fig. 4e and Roozendaal and Mebius [19] ), we sought to determine whether any of the known stromal cell subsets could be observed capturing and/or maintaining fluorescently labelled antigen at late time points after subunit vaccination. As we predicted from Fig. 4a , FDCs possessed little to no detectable antigen 6 days after vaccination ( Fig. 4e ). However, fluorescent antigen associated with LECs persisted for more than 3 weeks after vaccination ( Fig. 4f,g ). This apparent antigen capture by LECs was not related to the use of ovalbumin as a model antigen, as similar results were obtained with fluorescently labelled influenza nucleoprotein (NP) ( Supplementary Fig. 2 ). We further examined LECs and their capture of fluorescent antigen through the use of multi-photon microscopy 2 weeks after immunization with fluorescent antigen. To examine the localization of fluorescent antigen within the three-dimensional architecture of the LN, fluorescently labelled polyclonal T and B cells were transferred intravenously (i.v. ), along with subcutaneous injection of fluorophore-conjugated αLyve-1 antibody, into the immunized mice the day before LN excision and microscopy. This method effectively identified T-cell and B-cell regions, as well as the LECs lining the subcapsular sinus and the interfollicular ridges, respectively. Consistent with the flow cytometric data, fluorescently labelled antigen could be seen encapsulating the LN and branching into the interfollicular ridges where LECs reside, and indeed specifically co-localized with a portion of the αLyve-1 staining ( Fig. 4g and Supplementary Movie 1 ). Persisting antigen is not presented by LECs Given that LECs can present antigens to the naive T-cell pool [16] , we next examined whether or not the LECs were presenting the persisting vaccine-derived antigen directly to the circulating T cells. We initially used a pH-sensitive fluorophore-coupled antigen (ova-DQ) to investigate whether LEC-acquired antigen was endocytosed into endocytic compartments involved in antigen processing and presentation. Mice were vaccinated with either ova-AF488 or ova-DQ in combination with polyIC/CD40, and 1 week later the stromal cells were examined by flow cytometry for the amount of fluorescence derived from either antigen. As before, >50% of LECs were marked with the ova-AF488 antigen, indicating robust antigen capture. In contrast, ova-DQ fluorescence on LECs was minimal ( Fig. 5a ), suggesting that the majority of injected ova-DQ failed to access a late endosomal compartment. These data indicate one of two possibilities. First, the majority of persisting antigen is maintained either on the cell surface or within a non-lysosomal endocytic compartment. If correct, then LECs would not be expected to directly present antigen to circulating T cells. Second, persisting antigen may be so slowly taken up for processing that it provides only a minimal fluorescent signal with the DQ reagent. If correct, then LECs would be expected to directly present antigen to T cells. 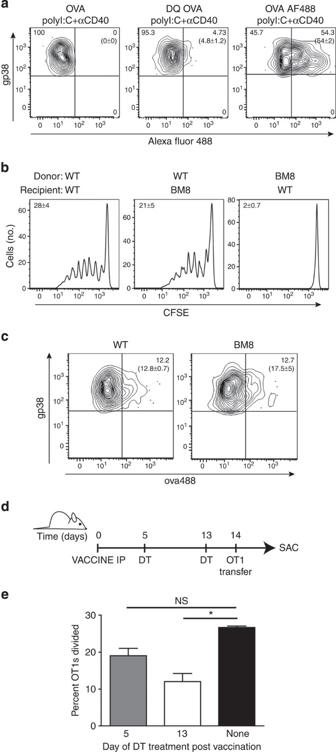Figure 5: Haematopoietically derived APCs are required for presenting persisting antigen to circulating T cells. (a) B6 mice were vaccinated with either ova-AF488 or ova-DQ+adjuvant as inFig. 4e. Seven days later, mice were killed and LEC fluorescent antigen capture (AF488) or LEC fluorescence (Ova-DQ) was determined by flow cytometry as described inFig. 4eand Methods. Numbers not in parentheses show the per cent of cells with in the region of that specific plot. Numbers in parentheses show the average per cent and s.e.m. of the per cent of cells within the region calculated from all mice in each group. (b) WT or BM8 recipient mice were lethally irradiated and reconstituted with either WT or BM8 donor bone marrow. Reconstituted mice were immunized with ovalbumin, polyI:C and αCD40, and 2 weeks post immunization, CFSE labelled OT1 T cells were transferred and monitored for CFSE dilution as inFig. 1. The average per cent dividing cells and s.e.m. of all mice in each group, calculated as described in Methods, are shown within each plot. (c) WT or BM8 mice were immunized and analysed for fluorescently labelled ova on LECs as inb. Numbers in plot are as ina. (d) Schematic representation of experimental method fore. Irradiated B6 mice reconstituted with CD11c-DTR bone marrow were injected with ova/polyI:C/anti-CD40 and at the indicated times post vaccination were injected with DT as described in the Methods. Fourteen days after vaccination, CFSE-labelled OT1s were transferred and monitored for division as inFig. 1. (e) Per cent OT1s divided from each treatment group was calculated as described in Methods. Significance was calculated using a Student’st-test. *P-value<0.05. Experiments were repeated at least twice with three mice per group with similar results. Figure 5: Haematopoietically derived APCs are required for presenting persisting antigen to circulating T cells. ( a ) B6 mice were vaccinated with either ova-AF488 or ova-DQ+adjuvant as in Fig. 4e . Seven days later, mice were killed and LEC fluorescent antigen capture (AF488) or LEC fluorescence (Ova-DQ) was determined by flow cytometry as described in Fig. 4e and Methods. Numbers not in parentheses show the per cent of cells with in the region of that specific plot. Numbers in parentheses show the average per cent and s.e.m. of the per cent of cells within the region calculated from all mice in each group. ( b ) WT or BM8 recipient mice were lethally irradiated and reconstituted with either WT or BM8 donor bone marrow. Reconstituted mice were immunized with ovalbumin, polyI:C and αCD40, and 2 weeks post immunization, CFSE labelled OT1 T cells were transferred and monitored for CFSE dilution as in Fig. 1 . The average per cent dividing cells and s.e.m. of all mice in each group, calculated as described in Methods, are shown within each plot. ( c ) WT or BM8 mice were immunized and analysed for fluorescently labelled ova on LECs as in b . Numbers in plot are as in a . ( d ) Schematic representation of experimental method for e . Irradiated B6 mice reconstituted with CD11c-DTR bone marrow were injected with ova/polyI:C/anti-CD40 and at the indicated times post vaccination were injected with DT as described in the Methods. Fourteen days after vaccination, CFSE-labelled OT1s were transferred and monitored for division as in Fig. 1 . ( e ) Per cent OT1s divided from each treatment group was calculated as described in Methods. Significance was calculated using a Student’s t -test. * P -value<0.05. Experiments were repeated at least twice with three mice per group with similar results. Full size image To distinguish between these two possibilities and address whether LECs could present captured antigen to circulating T cells, we used mice with a mutant form of MHC (K bm8 ), which cannot stimulate OT1 transgenic T cells with the SIINFEKL peptide [43] , [44] . Using bone marrow chimeras, we determined whether haematopoietic and/or non-haematopoietic cells could present persisting antigen. Following reconstitution of wild-type (WT) or K bm8 recipients with WT or K bm8 bone marrow, we observed that stimulation of T cells by persisting antigen required the presence of haematopoietic cells that can present the antigenic peptide ( Fig. 5b ). The persistence of fluorescent antigen could be detected on WT or K bm8 LECs ( Fig. 5c ). Thus, antigen is able to persist on LECs despite the inability of antigen to be presented. However, no proliferation of the transferred OT1 cells occurred in the WT mice reconstituted with K bm8 bone marrow ( Fig. 5b ), suggesting that even though antigen persists on LECs, it is not presented by LECs. These data indicated that although persisting antigen was harboured by the LECs, antigen presentation to T cells required the participation of cells of haematopoietic origin. DCs are critical to the response of naive T cells in the majority of experimental systems, and as such were the main haematopoietic cell type we expected to be involved in presenting persisting antigen. Indeed, previous studies documented a central role for DCs in presenting antigen persisting after viral infection [1] , [20] . We therefore used the CD11c-DTR mice, which express the diphtheria toxin (DT) receptor on DCs, allowing the deletion of DCs by administration of DT. Because of toxicity issues when using the intact CD11c-DTR host, we made chimeric mice by transferring bone marrow from CD11c-DTR mice into irradiated WT recipients. After reconstitution, mice were immunized with antigen and combined αCD40/polyI:C. DT was administered 5 or 13 days post immunization with a dose of DT determined to transiently deplete (for 24–48 h) >98% of all CD11c + cells from the secondary lymphoid tissue [23] . Fourteen days after immunization (9 or 1 day after DC depletion) TCR transgenic T cells were transferred into DT-treated and control hosts, and the extent of their proliferation was again used to identify the persistence of antigen ( Fig. 5d ). DC depletion 5 days after immunization (9 days before T-cell transfer) failed to reduce antigen persistence as measured by the per cent of transferred T-cell proliferation ( Fig. 5e ), confirming that DCs do not harbour the persisting antigen. In contrast, administration of DT 1 day before T-cell transfer resulted in a significant (~\n60–70%) reduction in the proliferation of the transferred T cells ( Fig. 5e ). Thus, consistent with previous data in viral antigen persistence, DCs play a central, although not exclusive, role in presenting the persisting antigen to circulating T cells. Collectively, we conclude that persistence of antigen on the LECs occurs independent of haematopoietically derived antigen-presenting cells (APCs). However, LECs do not directly stimulate T cells specific for the persisting antigen. Rather, haematopoietic cells in general, DCs in specific, are required for the presentation of persisting antigen to circulating antigen-specific CD8 T cells. Interestingly, these data also indicate that transfer of antigen between LECs and DCs or other APCs must occur for persisting antigen to be seen by circulating antigen-specific T cells. LEC antigen acquisition as a consequence of LEC division Consistent with our data using the OT1 transfer system ( Fig. 4 ), we observed capture of fluorescent antigen by LECs in both μMT and Cr2 −/− mice ( Fig. 6a ). We next examined whether antigen-specific T-cell responses were necessary for antigen persistence. We initially used a Rag −/− x gBT-1 TCR transgenic to address this question as this host possesses T cells but cannot mount an ovalbumin-specific response. Using both the adoptive transfer and fluorescently labelled antigen methods, it was clear that there was a dramatic defect in the Rag −/− xgBT-1 mice to support persisting antigen ( Fig. 6a ). However, closer examination of the LECs in this host revealed two interesting observations. First, in contrast to the WT hosts, both μMT and Rag −/− x gBT-1 mice had significantly fewer LECs than their WT counterparts ( Fig. 6b ). Second, LECs in WT and μMT mice responded to vaccination by expanding between three- to sixfold ( Fig. 6b ). This increase in LECs appeared to be the result of proliferation as noted by Ki67 staining ( Fig. 6c ). In contrast, LECs in the Rag −/− x gBT-1 host failed to expand after immunization ( Fig. 6b ). 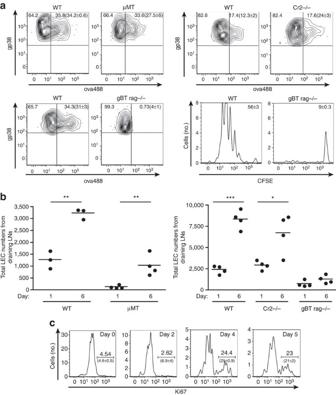Figure 6: Antigen persists only under conditions of LEC proliferation. (a) WT, μMT, gBT rag−/−mice were immunized with ova-488+polyI:C+anti-CD40, and 7 days later persisting antigen was measured by examining fluorescent antigen captured by LECs as inFig. 4e(for WT, Cr2−/−and gBT Rag−/−) and by CFSE dilution of labelled and transferred OT1 T cells as inFig. 1(for WT and gBT Rag−/−). Numbers not in parentheses show the per cent of cells with in the region of the specific plot. Numbers in parentheses show the average per cent and s.e.m. of the per cent of cells within the region calculated from all mice in each group. For CFSE dilution histograms, the numbers shown in each plot are calculated as inFig. 3. (b) Total numbers of LECs were calculated from draining LNs (axillary, brachial, inguinal and popliteal).P-values were calculated using Student’st-test where *P-value<0.05, **P-value<0.01 and ***P-value<0.001. (c) Mice were immunized as inaand killed on the indicated days. Draining LNs were prepared and stained for identification of Ki67 staining in LECs. Experiments were repeated at least twice with three to four mice per group with similar results. Average and s.e.m. from the experiment are shown in parentheses on the respective plot. Figure 6: Antigen persists only under conditions of LEC proliferation. ( a ) WT, μMT, gBT rag −/− mice were immunized with ova-488+polyI:C+anti-CD40, and 7 days later persisting antigen was measured by examining fluorescent antigen captured by LECs as in Fig. 4e (for WT, Cr2 −/− and gBT Rag −/− ) and by CFSE dilution of labelled and transferred OT1 T cells as in Fig. 1 (for WT and gBT Rag −/− ). Numbers not in parentheses show the per cent of cells with in the region of the specific plot. Numbers in parentheses show the average per cent and s.e.m. of the per cent of cells within the region calculated from all mice in each group. For CFSE dilution histograms, the numbers shown in each plot are calculated as in Fig. 3 . ( b ) Total numbers of LECs were calculated from draining LNs (axillary, brachial, inguinal and popliteal). P -values were calculated using Student’s t -test where * P -value<0.05, ** P -value<0.01 and *** P -value<0.001. ( c ) Mice were immunized as in a and killed on the indicated days. Draining LNs were prepared and stained for identification of Ki67 staining in LECs. Experiments were repeated at least twice with three to four mice per group with similar results. Average and s.e.m. from the experiment are shown in parentheses on the respective plot. Full size image T-cell expansion allows for LEC proliferation and archiving There are two possible explanations for the lack of antigen persistence in the Rag −/− x gBT-1 host: (i) an antigen-specific T-cell response is required for antigen acquisition/persistence by LECs, or (ii) LEC expansion/cell division, independent of the specificity of the T-cell response, is a necessary prerequisite to antigen acquisition/persistence. In this second possibility, vaccine-induced inflammation and the subsequent expansion of T cells within the draining LN would simply provide the necessary stimuli to the stroma to induce LEC proliferation via inflammation and/or baroreceptors. To distinguish between these possible mechanisms, we established a model that could track antigen persistence during a T-cell response in which the persisting antigen and responding T cells were unrelated. We transferred CD4 TCR transgenic T cells specific for the Eα-derived peptide 3K [45] into WT or Rag −/− x gBT-1 hosts. One day after CD4 T-cell transfer, mice were immunized with fluorescent ovalbumin with or without the 3K peptide. If the first model described above is correct (an antigen-specific T-cell response is required for the persistence of that antigen), then none of the Rag −/− x gBT-1 mice will demonstrate persistence of the ovalbumin antigen, as this host cannot mount any response to ovalbumin. However, if the second possibility is correct (any T-cell proliferation promotes antigen persistence), then the Rag −/− x gBT-1 hosts, which are co-immunized with the 3K peptide, will result in persistence of ovalbumin while the Rag −/− x gBT-1 hosts not immunized with 3K peptide will not. On analysis of the LECs 12 days after immunization, we observed that both WT and Rag −/− x gBT-1 hosts with expanded 3K-specific CD4 T cells captured fluorescent antigen ( Fig. 7a,b ), while the Rag −/− x gBT-1 mice not immunized with the 3K peptide failed to capture antigen. In addition, the number of LECs in the CD4-expanded Rag −/− x gBT-1 host proliferated to a similar degree as the LECs in the WT host ( Fig. 7c , 3K peptide). 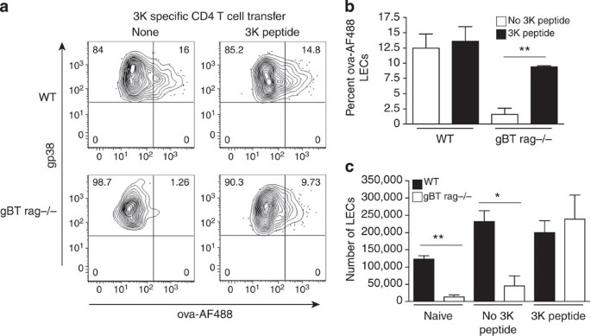Figure 7: Non-antigen specific T-cell expansion facilitates LEC proliferation and antigen archiving. (a) One thousand CD4 T cells from a 3K-specific CD4 T-cell transgenic mouse were transferred into WT or gBT rag−/−mice 12–18 h before immunization. Mice were left unimmunized or immunized subcutaneously with 10 μg ova-488+2 μg polyI:C+2 μg αCD40 (as above) ±3K peptide. Mice were killed 12 days post immunization and draining LNs prepared as inFig. 4. Shown are CD45−, CD31+, gp38+LECs. (b) Quantification ofa. (c) Total number of LECs expanded post immunization froma. Figure 7: Non-antigen specific T-cell expansion facilitates LEC proliferation and antigen archiving. ( a ) One thousand CD4 T cells from a 3K-specific CD4 T-cell transgenic mouse were transferred into WT or gBT rag −/− mice 12–18 h before immunization. Mice were left unimmunized or immunized subcutaneously with 10 μg ova-488+2 μg polyI:C+2 μg αCD40 (as above) ±3K peptide. Mice were killed 12 days post immunization and draining LNs prepared as in Fig. 4 . Shown are CD45 − , CD31 + , gp38 + LECs. ( b ) Quantification of a . ( c ) Total number of LECs expanded post immunization from a . Full size image Collectively, we conclude from these data that a T-cell response is a necessary component for inducing LEC expansion and subsequent antigen acquisition, not because of the specificity of the response, but because the expanding T cells promote the necessary stimuli to the stroma to induce LEC proliferation. These data support the model that LECs capture antigens involved in robust immune responses, in effect, ‘archiving’ them based on whether or not the ensuing immune response stimulated LECs to proliferate. Persisting antigen benefits CD8 + T cell protective memory Antigen persistence in viral model systems affects the functional status of circulating memory cells, increasing their effector functions and peripheral trafficking patterns [2] , [3] , [5] , [10] . We therefore established a model system in which we could interrogate the functional response of memory CD8 + T cells formed in the presence or absence of persisting antigen. As a source of effector/memory T cells, we isolated T cells from an ovalbumin-immunized, congenically marked (CD45.2) Vβ5 TCR transgenic host. These mice express only the TCRβ chain of the OT1 TCR (Vβ5), requiring the recombination of, and pairing with, endogenous TCRα chains. As a result, the T-cell repertoire has an elevated frequency of ova-specific T cells in the midst of a diverse repertoire of other specificities [46] . Besides the advantage of having a polyclonal response to ovalbumin, the Vβ5 transgenic host does not show any of the functional abnormalities sometimes associated with traditional TCR transgenic cells [47] . By using a modified version of the model described above, Rag −/− x gBT-1 (CD45.1) mice were transferred with 3K CD4 T cells and immunized with 3K peptide with and without whole ovalbumin ( Fig. 8a ). Two weeks after immunization, Vβ5 effector/memory T cells were transferred i.v. into the different recipients. Effectively, these T cells then circulated in animals with (3K+ova) and without (3K only) LEC-archived ovalbumin. The T cells were allowed 2 more weeks to complete memory formation in the presence or absence of persisting antigen (4 weeks after initial immunization) at which point all recipient mice were challenged with LM-ova. The phenotype and function of the transferred T cells were examined and bacterial loads in the spleen determined in each host. 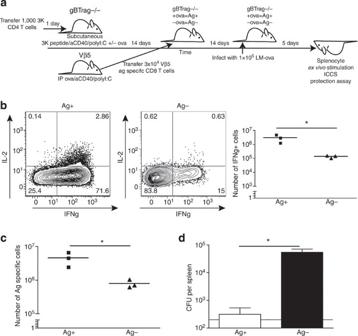Figure 8: Archived antigen enhances protective immunity. (a) Schematic of the experimental design forbandc. One thousand 3K- specific CD4 T cells were transferred 1 day before gBTxrag−/−mice. gBTxrag−/−(with 3K cells) were immunized subcutaneously with the 100 μg of the 3K peptide, 10 μg polyI:C and 10 μg αCD40±50 μg ovalbumin (as inFig. 6). Simultaneously, Vβ5 mice were immunized with 100 μg of ovalbumin, 50 μg aCD40 and 50 μg polyI:C. Two weeks later, CD8+T cells were isolated from the Vβ5 mice and 3 × 104SIINFEKL-specific CD8 cells/recipient were transferred into the previously immunized gBTxrag−/−mice with (Ag+) or without (Ag−) ovalbumin. Two weeks later mice were infected with 1 × 105LM-ova and 5 days after challenge, mice were killed and analysed for bacterial load and T-cell phenotype/function. (b) Spleen T cells from recipients described ina, stimulated directlyex vivowith SIINFEKL peptide in brefeldin A and stained for intracellular IFNγ and IL-2. Cells are gated on live, CD8+, B220−and CD45.1/2. Representative flow plots of the expression of IL-2 and IFNγ are shown with or without archived antigen. The number of IFNγ+cells are quantified in the right panel ofb. (c) The number of antigen-specific T cells from each mouse with archived or acute antigen exposure was calculated and plotted. (d) The number of colony-forming units (CFUs) was calculated per spleen on day 5 post infection. The limit of detection is displayed as a dotted line between 102and 103CFU. These experiments were repeated three times with three to four mice per group with similar results. Figure 8: Archived antigen enhances protective immunity. ( a ) Schematic of the experimental design for b and c . One thousand 3K- specific CD4 T cells were transferred 1 day before gBTxrag −/− mice. gBTxrag −/− (with 3K cells) were immunized subcutaneously with the 100 μg of the 3K peptide, 10 μg polyI:C and 10 μg αCD40±50 μg ovalbumin (as in Fig. 6 ). Simultaneously, Vβ5 mice were immunized with 100 μg of ovalbumin, 50 μg aCD40 and 50 μg polyI:C. Two weeks later, CD8 + T cells were isolated from the Vβ5 mice and 3 × 10 4 SIINFEKL-specific CD8 cells/recipient were transferred into the previously immunized gBTxrag −/− mice with (Ag + ) or without (Ag − ) ovalbumin. Two weeks later mice were infected with 1 × 10 5 LM-ova and 5 days after challenge, mice were killed and analysed for bacterial load and T-cell phenotype/function. ( b ) Spleen T cells from recipients described in a , stimulated directly ex vivo with SIINFEKL peptide in brefeldin A and stained for intracellular IFNγ and IL-2. Cells are gated on live, CD8 + , B220 − and CD45.1/2. Representative flow plots of the expression of IL-2 and IFNγ are shown with or without archived antigen. The number of IFNγ + cells are quantified in the right panel of b . ( c ) The number of antigen-specific T cells from each mouse with archived or acute antigen exposure was calculated and plotted. ( d ) The number of colony-forming units (CFUs) was calculated per spleen on day 5 post infection. The limit of detection is displayed as a dotted line between 10 2 and 10 3 CFU. These experiments were repeated three times with three to four mice per group with similar results. Full size image The transferred memory cells in the hosts with archived antigen showed increased interferon-γ (IFNγ) and interleukin-2 (IL-2) production after challenge with LM-ova as compared with memory T cells circulating in the hosts without archived antigen ( Fig. 8b ). Consistent with the increased IL-2 production of these cells, there was a greater expansion of the transferred T cells in the host with archived antigen compared with the host without archived antigen ( Fig. 8c ), despite similar frequencies of antigen-specific T cells before LM challenge ( Supplementary Fig. 3 ). Further, archived antigen had a dramatic impact on protection against LM challenge, promoting a two to three logs reduction in bacterial load ( Fig. 8d ). We conclude from these studies that LEC-archived antigen has a positive impact on the maintenance of protective CD8 T-cell memory by influencing the capacity of the circulating memory cells to expand in response to secondary challenge. Antigen archiving on LECs following vaccinia infection The mechanism by which antigen is captured and archived on LECs in our vaccine model system suggested that the same process should likely be involved during a viral infection. As mentioned above, stromal cell involvement in viral antigen persistence has been previously reported but has never ruled in or out any possible involvement of LECs. Indeed, challenge of both WT and CR2 −/− hosts showed that Vaccinia-derived antigen persisted equally well in both of these hosts ( Fig. 9a ), indicating that that FDC capture of antigen/antibody complexes is not responsible for antigen persistence following viral challenge. We therefore challenged mice with a strain of Vaccinia [48] expressing the Influenza NP protein conjugated to the fluorescent protein mCherry (NP-S-mCherry). Mice were infected in the footpad with NP-S-mCherry [48] or control VV-ova. To identify sites of viral replication/antigen, LN sections from infected mice were stained to visualize the LECs, subcapsular macrophages, and B cell follicles by confocal microscopy ( Fig. 9b ). At time points towards the end of viral replication within the node (3 days post infection [49] ), virus fluorescence was easily detected in close proximity to the subcapsular region and interfollicular ridges ( Fig. 9c,e ), consistent with previous reports [49] , [50] . Well after the clearance of actively replicating virus [49] , we observed a substantial reduction in the viral antigen fluorescence within the LN sections, as expected ( Fig. 9d ). However, the association of viral antigen fluorescence with LECs was dramatically enriched over time as determined by proximity of viral fluorescence to αLyve-1 staining ( Fig. 9d,e ). Thus, LECs appear to archive viral antigen for extended periods after viral challenge, indicating that LEC antigen capture and archiving is an active process for both infectious and vaccination settings. 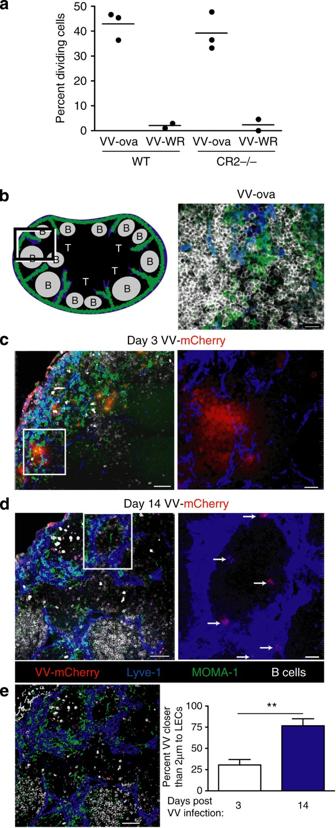Figure 9: Vaccinia-related antigen persists on LECs. (a) As inFig. 1, WT and Cr2−/−mice were challenged with VV-ova and antigen persistence was determined by transfer of CFSE-labelled OT1 cells at 18 days post infection. As shown and calculated inFig. 1, the data is expressed as per cent OT1 cells that divided 3 days after T-cell transfer. The per cent of OT1 cells that are dividing was calculated as described in the Methods. (b) Schematic and staining of a LN from a mouse infected withVaccinaexpressing ova (VV-ova) without the mCherry fluorophore. B cells are depicted in white, MOMA-1 subcapsular macrophages are depicted in green and Lyve-1+LECs are depicted in blue. Scale bar, 15 μm. (c) LN sections from mice 3 days after subcutaneous challenge with Vaccinia-NP-S-mCherry. VV-mCherry fluorescence is depicted in red. Scale bar, 50 μm. The white box indicates the area of the image analysed under higher magnification on the right. The higher magnification image shows only the Lyve-1 and VV-mCherry fluorescence. Scale bar, 10 μm. (d) LN sections from mice 14 days after subcutaneous challenge with Vaccinia-NP-S-mCherry, analysed as inb. Scale bar, 50 μm (in the left image) and 10 μm (at higher magnification). (e) Distance between Lyve-1 and mCherry fluorescence was calculated using the surface function in IMARIS. The image shown on the left demonstrates how the surfaces were made and the calculation on the right is the average of multiple images from at least three separate LNs. Scale bar, 50 μm (in the surface image). This experiment was repeated three times and images from multiple different LNs were taken. The data shown are representative images from each time point. Figure 9: Vaccinia-related antigen persists on LECs. ( a ) As in Fig. 1 , WT and Cr2 −/− mice were challenged with VV-ova and antigen persistence was determined by transfer of CFSE-labelled OT1 cells at 18 days post infection. As shown and calculated in Fig. 1 , the data is expressed as per cent OT1 cells that divided 3 days after T-cell transfer. The per cent of OT1 cells that are dividing was calculated as described in the Methods. ( b ) Schematic and staining of a LN from a mouse infected with Vaccina expressing ova (VV-ova) without the mCherry fluorophore. B cells are depicted in white, MOMA-1 subcapsular macrophages are depicted in green and Lyve-1 + LECs are depicted in blue. Scale bar, 15 μm. ( c ) LN sections from mice 3 days after subcutaneous challenge with Vaccinia-NP-S-mCherry. VV-mCherry fluorescence is depicted in red. Scale bar, 50 μm. The white box indicates the area of the image analysed under higher magnification on the right. The higher magnification image shows only the Lyve-1 and VV-mCherry fluorescence. Scale bar, 10 μm. ( d ) LN sections from mice 14 days after subcutaneous challenge with Vaccinia-NP-S-mCherry, analysed as in b . Scale bar, 50 μm (in the left image) and 10 μm (at higher magnification). ( e ) Distance between Lyve-1 and mCherry fluorescence was calculated using the surface function in IMARIS. The image shown on the left demonstrates how the surfaces were made and the calculation on the right is the average of multiple images from at least three separate LNs. Scale bar, 50 μm (in the surface image). This experiment was repeated three times and images from multiple different LNs were taken. The data shown are representative images from each time point. Full size image Our data demonstrate an unexpected role for LECs in harbouring antigen following the induction of cellular immunity in response to vaccination or viral challenge. The capture/archiving of persisting antigen by this stromal cell requires a productive T-cell response but is independent of the responding T-cell specificity, instead coinciding with LEC proliferation within the local lymphoid tissue. These results present a novel mechanism by which the local secondary lymphoid tissue stroma can sense the degree of local inflammation and archive antigens against which a strong immune response has been generated. Although antigen persistence after infectious challenge is well documented [1] , [2] , [3] , [4] , [5] , our data show for the first time that vaccination can also lead to persistence of antigen for periods of time well beyond the rise and fall of the T-cell response. Our data is also the first to demonstrate that LECs can serve as a reservoir for antigen that can be subsequently presented to antigen-specific CD8 T cells by haematopoietically derived APCs, in turn leading to increased effector function and immune protection by circulating memory CD8 T cells. It is necessary to contrast the antigen persistence observed in our data, as well as in the infectious models discussed above, from the high levels of antigen observed following some chronic viral infections and vaccine-related antigen depots. Although both result in the maintenance of antigen within the host for extended periods of time after the peak adaptive response, differences in the location of the antigen seem to correlate with the vastly different effects each type of persisting antigen has on the development of protective immune memory. Chronic viral infections (such as LCMV clone13) produce high levels of antigen that persists within the peripheral tissues as well as within lymphoid tissues. In these cases, the T-cell response ultimately suffers from tolerance mediated by clonal exhaustion [51] . In contrast, antigen persistence in response to acute viral infections (influenza, vaccinia), or subunit vaccination as we show here, is largely, if not exclusively, localized within the secondary lymphoid organs (SLO). Data from the viral models show that this SLO-associated antigen periodically stimulates circulating memory cells to proliferate and/or differentiate into more effector-like cells [2] , [3] , [5] , [10] , enhancing the trafficking of antigen-specific cells into the peripheral tissues and ultimately promoting more immediate protection against potential re-infection [1] , [2] , [3] , [4] , [5] . Consistent with this, we found an increase in the number of IL-2 + IFNγ + cells and an increased protection against bacterial challenge in mice with archived antigen. Collectively, the data suggest that chronic peripheral (non-lymphoid tissue) sites of antigen deposition are detrimental to the development and/or maintenance of immune memory, while SLO sites of antigen promote protective memory by modulating the differentiation status of the circulating memory pool. An important confirmation of this prediction is seen in the detrimental effect that vaccine emulsions can have on the magnitude/maintenance of immune memory. We [52] and others [53] , [54] have shown that the immune memory derived from subunit vaccination can all be eliminated by simply formulating the vaccine into an emulsion [52] , [53] . A recent publication by Hailemichael et al. [54] elegantly shows how the emulsion forms a peripheral antigen depot that sequesters effector/memory cells, inducing their dysfunction and deletion. This is consistent with older data on antigen-specific CD4 + T cells and their tendency to localize in the injection site [55] . Thus, chronic viral infections and vaccine emulsion antigen depots have a similar negative impact on productive immune memory, likely to be through a common mechanism of tolerance/deletion enforced by long-lived antigen deposition within a peripheral tissue. Ultimately, these data indicate that a better delineation between the various forms of antigen persistence within the vaccinated/challenged host is necessary. We propose the term ‘antigen archive’ to describe residual antigen that persists within the SLO following vaccination or acute infection. An archive can be loosely defined as an active process by which material or data is preserved, a definition that matches well with the various observations of antigen capture and maintenance by SLO stromal cells. In this regard, our documentation of a central role for proliferating LECs in antigen archiving is both highly unexpected and significant. Previous work investigating how antigen persists showed necessary functions for the B-cell follicle, FDCs and/or antigen antibody complexes in long-term antigen persistence [1] , [36] , [40] , [56] . A broad diversity of model systems, from infections to pregnancy, have documented various mechanisms by which FDCs capture and archive antigen for future B- and T-cell stimulation [36] , [57] , [58] , [59] , [60] . Indeed we anticipated FDCs as the repository of archived antigen in our model system as well, making our demonstration of LECs as the antigen archive following subunit vaccination all the more significant. Perhaps even more surprising is the role for LEC proliferation in the process of archiving antigen. It is as of yet unclear what specific signals are required to induce LEC proliferation in the context of vaccination and viral infection. Our data indicate that inflammation ( Fig. 2 ) and T-cell expansion ( Fig. 7 ) are both necessary to induce LEC proliferation. The simplest model would suggest that these signals are perhaps necessary only to promote LN swelling, which signals through baroreceptors to stimulate LEC proliferation to keep up with the growing size of the SLO. However, the data resulting from vaccination using αCD40 alone, or with LM infection, suggests a more complex model. Anti-CD40 vaccination of the host typically results in expansion of B cells in the SLO, not to mention a degree of T-cell expansion that is typically greater than that seen in response to other single adjuvants [21] , [22] , [27] . Further, LM challenge clearly elicits robust CD4 and CD8 + T-cell immunity in the presence of numerous inflammatory signals. However, neither promotes antigen archiving nearly to the degree that viral challenge or polyI:C do ( Figs. 1 , 2 and 3 ), indicating more specific signals are required for inducing antigen archiving than LN swelling alone. Given the propensity for antigen to persist following viral challenge and not bacterial, there may be additional requirements for direct activation of the stromal cells by the adjuvant/virus via specific innate receptors to induce antigen capture by LECs [17] , [61] , [62] . LECs have been shown to tolerize tumour/self-specific CD8 T cells by presenting self antigen [15] , [16] , [18] , [19] , [63] . We were therefore somewhat surprised at the inability of the LECs to present archived antigen to circulating T cells ( Fig. 5 ). However, given the fact that only limited subsets of professional APCs are capable of MHC class I presentation of exogenous antigens (cross presentation) [64] , [65] , [66] , [67] , perhaps it is not surprising that the LECs can only present endogenous/self antigens via class I MHC but not the exogenously provided vaccine/viral antigens. The requirement for haematopoietic cells in the presentation of persisting antigen indicates that some form of antigen transfer between the LECs and the APC must occur, perhaps similar to that observed between different DC subsets [68] , or FDCs and DCs [36] . How and in what form the antigen might be captured and maintained is as yet undetermined. Our use of DQ-coupled antigen indicates that little of the retained antigen finds it’s way into late endosomal compartments ( Fig. 5a ), suggesting that the retained antigen may be surface bound or perhaps involved in a form of recycling of surface-bound antigen as has been recently demonstrated for FDCs [12] . Antigen transfer between B cells and FDCs has been previously shown to involve CR1/2, which are not expressed on LECs [19] , [40] . Whatever the mechanisms of antigen transfer, DCs are clearly responsible for the majority, although not all, of the presentation of the persisting antigen that is archived by the LECs ( Fig. 5 ). A reasonable prediction is that DCs from the peripheral tissues acquire antigen from the LECs as they migrate through the interfollicular ridges and into the T-cell zones of the local node. The molecular means by which the proliferating LECs capture and hold antigen and the long-term impact on vaccine-elicited cellular immunity is the focus of future work. Mice In general, 6-to 8-week-old female WT, BM8, gBT-1 rag −/− , μMT, MHC classII −/− , Cr2 −/− , MD4, 3K, rag −/− OT1 and Vβ5 mice were all bred on a C57bl/6 background. Mice were purchased from either the National Cancer Institute or The Jackson Laboratory, unless otherwise stated, and bred in house. Cr2 −/− mice were a kind gift from Michael Holers laboratory at the University of Colorado, Denver, CO. OT1 mice are a TCR transgenic strain specific to the SIINFEKL peptide of ovalbumin (OVA257-264) in the context of H-2K b . β mice only express the transgene for the β-chain of the OT1 TCR. Normal thymic selection at the α-chain leads to a diverse repertoire that has 1–3% ova-specific CD8 + T cells. gBT-1 (gBT) mice (a kind gift from Bill Heath, University of Melbourne) are a TCR transgenic strain specific to the SSIEFARL peptide of herpes simplex virus glycoprotein B, HSV-1 gB 498–505 in the context of H-2K b . 3K mice are a TCR transgenic specific to the 3K peptide, which is a variant of the Ea peptide in the context of IA b (ref. 45 ). These mice were a kind gift from the Kappler/Marrack lab at the National Jewish Health, Denver, CO. B6.C-H-2K bm8 (BM8) H-2K b mutant cannot effectively present the SIINFEKL peptide to OT1 T cells to induce T cell activation. BM8 mice were a kind gift from Larry Pease, Mayo Foundation, Rochester, MN. MD4 mice are an IgMα B-cell receptor transgenic strain specific to hen egg lysozyme. MD4 mice were a kind gift from John Cambier, University of Colorado, Denver, CO. All animal procedures were approved by the Institutional Animal Care and Use Committee at National Jewish Health. Stromal and DC harvesting and staining Mice were immunized subcutaneously with 0–20 μg of antigen (ova-AF488 or ova-DQ (Life Technologies)) with 2 μg polyI:C and 2 μg αCD40 (per site) into five sites (footpads, flanks, scruff). Mice were killed at 1–21 days, and popliteal, inguinal, axillary and brachial LNs were harvested into EHAA media without L -glutamine (GIBCO, Grand Island, NY). LNs were dissected using 22-guage needles to separate the tissue. Tissue was digested using 0.25 mg of Liberase DL (Roche, Indianapolis, IN) per ml of EHAA media and DNAse (Worthington, Lakewood, NJ) for 1 h at 37 °C. An equal volume of 0.1 M EDTA in Hank’s buffered saline solution without calcium or magnesium was added and incubated for 5 min at 37 °. Digested LNs were then pushed through a screen and washed with 5 mM EDTA in EHAA. All flow cytometry antibodies were purchased from Biolegend (San Diego, CA) unless otherwise stated. Stromal cells were stained with CD45 Pacific Blue clone 30-F11 (1:300), Gp38/podoplanin APC clone 8.1.1 (1:200), CD31 PerCp/Cy5.5 clone 390 (1:200) and CD21/35 phycoerythrin (PE) clone 7E9 (1:200). As published [19] , stromal cell subsets were identified as follows: blood endothelial cells, CD45 − gp38 − CD31 + ; LECs, CD45 − gp38 + CD31 + CD21/35 − ; FDCs, CD45 − gp38 + CD31 − CD21/35 + ; fibroblastic reticular cells and MRCs CD45 − gp38 + CD31 − CD21/35 − . DCs were stained with CD11c APC/Cy7 clone N418 (1:400), B220 PE clone RA3-6B2 (1:300), CD8 PerCP/Cy5.5 clone 53-67 (1:200) and CD11b Pacific Blue clone M1/70 (1:750) (eBioscience, San Diego, CA). DCs shown are gated on live, CD11c + , B220 − , and CD8 + CD11b − or CD8 − CD11b + cells. Cells were run on the DakoCytomation CyAn ADP flow cytometer (Fort Collins, CO) and acquired using Summit acquisition software. FlowJo software (Tree Star, Ashland, OR) was used to analyse flow cytometry data and cells were counted using a ViCell (Beckman Coulter, Brea, CA). Protection assay Approximately 1,000 3K CD4 T cells were transferred i.v. into gBT rag −/− mice (CD45.1). Cells were allowed to ‘park’ overnight before immunizing with 100 μg 3K peptide (ASFEAQ K A K AN K AVDKA)+10 μg polyI:C+10 μg anti-CD40 ±50 μg ovalbumin protein per mouse divided into the flanks, scruff and footpads. The same day Vβ5 (CD45.2) mice were immunized with 100 μg ovalbumin+50 μg polyI:C+50 μg anti-CD40. Immunization of Vβ5 with ovalbumin produces a substantial pool of memory cells within a diverse background of other specificities. Two weeks later the Vβ5 mouse was killed and CD8 T cells were isolated from the spleen and LNs using the STEMCELL CD8 T-cell isolation kit. Isolated CD8s were stained with antibodies against CD8 APC-Cy7 (Biolegend clon 53-6.7 1:600), CD45.1 PerCP Cy5.5 (Biolegend, clone A20 1:200), CD45.2 APC (Biolegend, clone 104 1:200), CD44 Pacific Blue (Biolegend, clone IM7 1:400) and SIINFEKL-specific tetramer (PE in house 1:200). SIINFEKL-specific T cells (3 × 10 4 ) were transferred i.v. into each mouse. Two weeks post CD8 T-cell transfer mice were challenged with 1 × 10 5 LM expressing the ovalbumin protein. After 4.5–5 days of LM challenge, mice were killed and spleens were cut in half. Half of the spleen was placed into 10 ml of 0.2% Igepal CA 630 (Sigma) and dissociated using a tissue grinder. Ground spleens were diluted in PBS. All dilutions were plated onto BHI (Bacto-Brain Heart Infusion-BD) media with 5 μg ml −1 erythromycin (Sigma) for LM-ova selection. Plates were incubated at 37 °C for 2 days and colonies were counted. The other half of the spleen was placed into complete media and macerated with glass slides, red blood cells (RBCs) were lysed and the single-cell suspension was stimulated in Brefeldin A with or without the SIINFEKL peptide for 4 h at 37 °C. After stimulation, cells were stained with Biolegend antibodies: CD8 APC-Cy7 (clone53-6.7 1:600), B220 AF488 (clone RA3-6B2 1:300), CD45.1 PerCP Cy5.5 (clone A20 1:200) and CD45.2 Brilliant Violet (clone 104 1:200). Cells were fixed with 1% paraformaldehyde in 4% sucrose for 10 min and washed twice with FACs buffer. Cell membranes were then permeabilized with perm wash (BD) and intracellular cytokines IL2 PE (clone JE56-5H4 1:100) and IFNγ APC (clone XMG1.2 1:100) were used to stain cells overnight in perm wash. Cells were washed and run on the flow cytometer as described above. OT1 transfer assays Mice were immunized 1–30 days before OT1 T cell transfer. CD45.1 congenically marked OT1 T cells were isolated by negative selection using the Miltenyi (Miltenyi, Auburn, CA) or Stem Cell Technologies’ (Vancouver, BC) CD8-negative selection kits. Greater than 90% CD8 T-cell purity was obtained by either method. Following negative selection, OT1s were labelled with CFSE or Violet Proliferation Dye (VPD; Invitrogen) and 2 × 10 5 –1 × 10 6 labelled T cells were transferred into immunized C57bl/6 mice (CD45.2). Three days post transfer mice were killed, and spleens and draining LNs were harvested. Tissues were macerated with glass slides, RBC lysed with ACK buffer and stained with CD45.1, CD45.2, B220, CD8, CD44, and SIINFEKL-specific tetramer (as above) to assess transferred OT1 T-cell proliferation. Determination of the fraction of cells that have divided at least once (per cent dividing cells) was calculated as previously described [69] using the equation fraction diluted=∑ i 1 N i /2 i /∑ i 0 N i /2 i , where i is the generation number (0 is the undivided population) and N i is the number of events in generation i . Vaccines and pathogen challenge Draining LNs and spleen were used to gather activated T cells. Ovalbumin (Sigma-Aldrich, St. Louis, MO) or HSVgB (produced in the lab using baculovirus expression) were decontaminated of lipopolysaccharide using a Triton X-114 lipopolysaccharide detoxification method [70] , used in combination with polyI:C (GE Healthcare), pam3CSK4 [N-palmitoyl- S -2,3-bis(palmitoyloxy)-(2R,S)-propyl]-(R)-cysteine-(S)serine-(S)lysine 4] (InvivoGen, San Diego, CA), anti-CD40 (clone FGK4.5, BioXCell, West Lebanon, NH) or the TLR7a agonist, 3M012, conjugated to ovalbumin [32] , [33] . For pathogen challenge, female B6 mice were injected with either 1 × 10 7 pfu per mouse of VV Western Reserve Strain expressing the ovalbumin protein (VV-ova) or 1 × 10 5 LM expressing whole ovalbumin protein (LM-ova). Bone marrow chimeras WT or BM8 mice were irradiated with 900 rads and rested for 4 h before reconstitution with either WT, BM8, or CD11c-DTR bone marrow. Bone marrow was isolated and RBCs were lysed before i.v. transfer. At 12 weeks post reconstitution, mice were immunized as described above. For CD11c DTR experiments, mice were vaccinated and 100 ng of DT (Sigma-Aldrich) was injected intraperitoneally at the indicated time points as previously described [23] . Multi-photon microscopy Multi-photon imaging was done using an Olympus FV1000MPE microscope with a XLPLN25XWMP Super 25 × 1.05 numerical aperture water-immersion objective and a Spectra Physics 10-W Mai-Tai DeepSee-OL laser. Bulk T cells were purified as described above with a Miltenyi column and labelled with VPD (BD Biosciences) for 25 min at 37 °C and washed. Bulk B cells were purified using negative selection with PE-conjugated antibodies (0.014 μl per 10 6 cells) to CD3 (Biolegend, clone 145-2C11), CD4 (BD Pharmingen, clone GK1.5), CD8 (eBioscience, clone 53-6.7), CD11c (Biolegend, clone N418), CD11b (BD Pharmingen M1/70), NK1.1 (Biolegend, clone DK136), IA/IE (Biolegend, clone M5/114) and CD49d (Biolegend, clone DX5). Cells were bound to anti-PE magnetic beads and run over a Miltenyl LS column and the flow through was taken. The purified B cells were labelled with CMTMR (Invitrogen) for 25 min at 37 °C and washed. Total B and T cells (5 × 10 6 )were injected i.v. into mice 12–18 h before imaging. Two to five micrograms of αLyve-1 conjugated to AlexaFluor 647 was injected subcutaneously into the footpad of immunized and transferred mice 12–18 h before imaging. Popliteal LNs were excised and fat was removed. Explanted LNs were immobilized to coverslips with efferent lymphatics adhered to coverslips. A 3 × 3 grid of Z -stack images with each XY plane spanning 509 μm × 509 μm at a resolution of 0.994 μm per pixel was acquired to encompass the whole LN. Each Z -stack covered a total depth of 300 μm in 5 μm Z -step increments. T-cell VPD fluorescence was captured by the 450–490 nm filter, ovalbumin conjugated to Alexa Fluor 488 was captured by the 500–550 nm filter, B-cell CMTMR fluorescence was captured by the 575–640 nm filter and Lyve-1 Alexa Fluor 647 was captured by the 645–685 filter for channel acquisition. Analysis of LN Z -stack images was done using Xuv stitch GUI 1.8.099 × 64.Ink software to reassemble together the nine images taken from the explanted LN to visualize the entire node. The channel arithmetics function in the Imaris software (Bitplane) was used to compensate between colours on the LN images with no antigen. The same settings were used for LN images from the antigen-immunized mice that were calculated using the control naive mouse. Using the co-localization function in Imaris, Lyve-1 and antigen co-staining were made into a new channel and visualized as yellow. Confocal microscopy Mice were infected with 1 × 10 5 VV-ova or VV-NP-S-mcherrry (Yewdell) subcutaneously in the footpad 3 or 14 days before killing. Popliteal LNs were harvested from infected mice and fixed for 45 min in 1% paraformaldehyde before imbedding the node into OCT (optimal cutting temperature) compound. Ten-micrometre sections were cut using a cryostat and stained with Lyve-1 (R&D systems) either directly conjugated to AF647 (Invitrogen, 1:50) or αLyve-1 biotin (R&D systems, 1:100) followed by strepavidin pacific blue (R&D systems, 1:500), MOMA-1 fluorescein isothiocyanate (AbC Serotec, clone MCA947F 1:50) and B220 biotin (BD Pharmingen, RA3-6B2 1:100) followed by strepavidin pacific blue or IgM AF650 (a kind gift from Raul Torres, clone R33.24.12 1:100). Sections were imaged using a Zeiss LSM 700 confocal microscope at × 40 magnification. For VVmCherry-infected nodes, 3 × 3 scans were acquired with ~\n20 0.5 μm Z -sections. Images were analysed using Imaris software as described above. Following channel arithmetics, surface masks were created for LECs, B cells and VV-associated mcherry fluorescence. The number of mcherry surfaces <2 μm from other created surfaces was calculated using a script created in Matlab (Mathworks). Multiple LN sections were analysed from five LNs of infected mice. Statistical analysis Statistical analysis was done using the Student’s t -test in prism4 (GraphPad, San Diego, CA). * P -value <0.05 and ** P -value <0.01. Each analysis was done with at least three mice per group and each experiment was done at least twice with the same results. How to cite this article: Tamburini, B. A. et al. Antigen capture and archiving by lymphatic endothelial cells following vaccination or viral infection. Nat. Commun. 5:3989 doi: 10.1038/ncomms4989 (2014).